Identification of a phosphorylation site on Ulk1 required for genotoxic stress-induced alternative autophagy Alternative autophagy is an autophagy-related protein 5 (Atg5)-independent type of macroautophagy. Unc51-like kinase 1 (Ulk1) is an essential initiator not only for Atg5-dependent canonical autophagy but also for alternative autophagy. However, the mechanism as to how Ulk1 differentially regulates both types of autophagy has remained unclear. In this study, we identify a phosphorylation site of Ulk1 at Ser 746 , which is phosphorylated during genotoxic stress-induced alternative autophagy. Phospho-Ulk1 746 localizes exclusively on the Golgi and is required for alternative autophagy, but not canonical autophagy. We also identify receptor-interacting protein kinase 3 (RIPK3) as the kinase responsible for genotoxic stress-induced Ulk1 746 phosphorylation, because RIPK3 interacts with and phosphorylates Ulk1 at Ser 746 , and loss of RIPK3 abolishes Ulk1 746 phosphorylation. These findings indicate that RIPK3-dependent Ulk1 746 phosphorylation on the Golgi plays a pivotal role in genotoxic stress-induced alternative autophagy. Macroautophagy (hereafter referred to as autophagy) is a catabolic process in which cellular contents are degraded [1] , [2] . Autophagy plays a pivotal role in a wide variety of physiological and pathological situations. The molecular basis of starvation-induced autophagy has been extensively studied, in which autophagic membranes originate from the endoplasmic reticulum (ER) or mitochondria-associated ER membrane and functional complexes containing autophagy-related (Atg) proteins drive the formation of autophagosomes [2] , [3] . Atg proteins are categorized into the following five functional groups: Unc-51 like autophagy activating kinase (Ulk1) and its regulators, the class III lipid kinases producing phosphatidylinositol 3-phosphate (PI3K), Atg9 complexes, the Atg5 conjugation system, and the microtubule-associated protein light chain 3 (LC3) conjugation system. After their generation, autophagosomes fuse with lysosomes to form autolysosomes by a mechanism dependent on syntaxin 17 (Stx17) [4] . In addition to this canonical autophagy, several types of noncanonical autophagy have been reported [5] , [6] , [7] . Atg5-independent alternative macroautophagy (hereafter described as alternative autophagy), which we discovered previously [5] , is one such type of autophagy. This autophagy machinery is also named Golgi membrane‐associated degradation (GOMED) [8] . Unlike canonical autophagy, autophagosomal membranes are derived from the trans -Golgi membrane [5] , [8] in alternative autophagy, and the mechanism involves Ulk1 and PI3K complexes, but not Atg9 complexes, Stx17 [9] , nor the Atg5 or LC3 conjugation system. Canonical and alterative autophagy are used differently in a stimulus/context-dependent manner, i.e., starvation induces mostly canonical autophagy, whereas genotoxic stress induces both canonical and alternative autophagy [5] . Furthermore, in the terminal differentiation of erythrocytes, alternative and canonical autophagy eliminate different substrates, i.e., mitochondria and ribosomes, respectively [10] . Despite morphological similarities, molecules involved in canonical and alternative autophagy are mostly different. However, Ulk1 is a serine/threonine kinase and a homolog of yeast Atg1 that is involved in both pathways at the initial step [5] , [10] . Ulk1 contains various phosphorylation sites, and their phosphorylation status regulates canonical autophagy [3] . Under unstimulated conditions, Ulk1 is phosphorylated at Ser 637 (amino acid residues are described according to mouse Ulk1, unless otherwise described) and Ser 757 by mammalian target of rapamycin complex 1 [11] , [12] , by which Ulk1 is inactivated. Upon starvation and genotoxic stress, Ulk1 is dephosphorylated at Ser 637 by protein phosphatase 2A [13] and protein phosphatase, Mg 2+ /Mn 2+ -dependent 1D (PPM1D) [14] , respectively. This dephosphorylation facilitates Ulk1 translocation to preautophagosomal membranes and activates its kinase activity, both of which are required for the induction of canonical autophagy. AMP-activated protein kinase (AMPK) was also reported to phosphorylate Ulk1 at Ser 317 , Ser 467 , Ser 555 , Ser 777 , and Thr 574 upon starvation [3] , [12] , [15] , [16] . Insulin-Akt signaling also induces Ulk1 phosphorylation at Ser 774 and blocks rapamycin-induced autophagy [16] . Thus, Ulk1 activity is regulated by the status of its multiple phosphorylation sites. Because more than 70 phosphorylation sites have been reported in Ulk1, additional kinases are expected to be involved in the regulation of Ulk1 activity and the resulting cellular events. In the mechanism of alternative autophagy, Ulk1 functions at the initial step [5] , [10] , because knockdown of Ulk1 suppressed the generation of isolation membranes. Unlike canonical autophagy, however, the mechanism of Ulk1 activation remains unclear. Therefore, to address this issue, we search for Ulk1 phosphorylation sites required for the induction of alternative autophagy. In this study, we identiy a phosphorylation site of Ulk1 at Ser 746 , which is required for the initial step of alternative autophagy, but not canonical autophagy, upon stimulation of genotoxic stress. We further identify receptor-interacting serine-threonine kinase 3 (RIPK3) as the kinase responsible for Ulk1 phosphorylation at Ser 746 . We also find that Ulk1 phosphorylated on Ser 746 is localized on the Golgi, where isolation membranes are generated. Taken together, these data indicate that RIPK3-dependent Ulk1 phosphorylation at Ser 746 is required for alternative autophagy, but not canonical autophagy. DNA damage induces Ulk1 phosphorylation at Ser 746 Ulk1 is a crucial molecule not only for canonical autophagy but also for alternative autophagy [5] . Unlike canonical autophagy, how Ulk1 is activated during alternative autophagy remains unknown. Because the properties and functions of Ulk1 are largely dependent on the phosphorylation status of each amino acid residue, we first investigated the sites of Ulk1 phosphorylation during alternative autophagy induced by etoposide, a DNA-damaging reagent and strong inducer of alternative autophagy. To this end, Ulk1 was immunoprecipitated with an anti-Ulk1 antibody from untreated and etoposide-treated Atg5 knockout (hereafter referred to as Atg5 KO ) mouse embryonic fibroblasts (MEFs), digested with trypsin, and then analyzed by LC–MS/MS. We detected various reported phosphorylation sites of Ulk1, such as Ser 317 , which is an AMPK target that is known to be phosphorylated during alternative autophagy [17] . In addition, we identified phosphorylation sites of Ulk1 at Thr 10 , Ser 297 , Ser 300 , Ser 302 , and Ser 783 in untreated Atg5 KO MEFs, and at Ser 308 , Ser 314 , Ser 494 , and Ser 746 in etoposide-treated Atg5 KO MEFs. Among these phosphorylation sites, we focused on Ser 746 (Fig. 1a ), because when various phosphodeficient Ulk1 mutants were expressed at equivalent levels in Atg5/Ulk1 double-knockout ( Atg5/Ulk1 DKO ) MEFs (Supplementary Fig. 1a, b ), most Ulk1 mutants, but not mutant Ulk1 (S746A), recovered the ability to perform alternative autophagy (Supplementary Fig. 1c, d ). The Ser 746 residue (corresponding to Ser 747 of human Ulk1) is conserved in Ulk1, but not Ulk2, of higher vertebrates (Supplementary Fig. 1e ). To analyze the role of Ulk1 phosphorylated at Ser 746 (p-Ulk1 746 ), we generated a specific antibody against p-Ulk1 746 that could be used for immunostaining and immunoprecipitation, but not for western blotting. To confirm the phosphorylation of Ser 746 of Ulk1 upon etoposide treatment, we immunoprecipitated p-Ulk1 746 using its specific antibody and analyzed the amount of precipitation by western blotting using an anti-Ulk1 antibody. As indicated, the level of endogenous p-Ulk1 746 was increased in Atg5 KO MEFs, but not in Atg5 / Ulk1 DKO MEFs, upon etoposide treatment (Fig. 1b ). The p-Ulk1 746 signal was completely abolished by the addition of recombinant phosphatase during the immunoprecipitation (Supplementary Fig. 2 ), indicating that the immunoprecipitation occurred in a phosphorylation-dependent manner. When we expressed HA-Ulk1 (wild-type; WT) in Atg5 / Ulk1 DKO MEFs, exogenous p-Ulk1 746 signals were also increased, whereas it was not observed upon the expression of the S746A phosphodeficient mutant (Fig. 1c ), despite mutant Ulk1 being expressed at a higher level than HA-Ulk1 (WT) (Fig. 1c ). These data validate the quality of the p-Ulk1 746 -specific antibody and confirmed the etoposide-induced phosphorylation of Ulk1 at Ser 746 . Note that a mobility shift in Ulk1 was observed in etoposide-treated cells on SDS–PAGE (Fig. 1b, c ), which might be due to the dephosphorylation of Ulk1 at other residues, such as Ser 637 , as previously described [14] . Analysis of Ser 637 dephosphorylation is described later. Fig. 1: Phosphorylation of Ulk1 at Ser 746 and its Golgi localization upon etoposide treatment. a Identification of an Ulk1 phosphorylation site. Ulk1 was immunoprecipitated with the anti-Ulk1 antibody from etoposide-treated Atg5 KO MEFs and subjected to trypsin digestion. The tryptic digests were analyzed by LC–MS/MS. This mass spectrum yielded a fragment ion spectrum displaying three C-terminal fragment ions (y-type) and seven N-terminal fragment ions (b-type). The result that y5-y4 is about 167 Da, which is equivalent to a phosphoserine, and database searching identified this peptide as TLHPGARGGGAS[Pho]SPAP, the partial sequence (amino acids 735–750) of the Ulk1 protein. b , c Phosphorylation of Ulk1 at Ser 746 by etoposide treatment. The indicated MEFs were treated with 10 µM of etoposide for the indicated times, lysed, and immunoprecipitated with an anti-p-Ulk1 746 antibody. Immune complexes and total lysates (2.8% input) were analyzed by western blotting using an anti-Ulk1 antibody. d , e Induction of the Golgi localization of p-Ulk1 746 by etoposide treatment. The indicated MEFs were treated with or without 10 µM of etoposide for 12 h, and immunostained with anti-p-Ulk1 746 and anti-GS28 antibodies. Nuclei were counterstained with Hoechst 33342 (50 ng mL −1 ). Representative images of p-Ulk1 746 (green; upper panels) and merged images (lower panels) of p-Ulk1 746 (green), GS28 (red), and Hoechst 33342 (blue) are shown. Magnified images of the areas within the dashed squares are shown in the inset. Arrowheads indicate p-Ulk1 746 signals. f Quantification of cells displaying p-Ulk1 746 signals. The indicated MEFs were treated with 10 µM of etoposide for the indicated times, and immunostained with an anti-p-Ulk1 746 antibody. The population of cells with p-Ulk1 746 signals was calculated ( n ≥ 100 cells in each experiment). Data are shown as the mean ± SD ( n = 3). Atg5/Ulk1 DKO + HA-Ulk1 (WT) no treatment vs. etoposide: p = 0.0002. Other exact p values cannot be described since the value is too large ( p > 0.9999) or small ( p < 0.0001). Comparisons were performed using one-way ANOVA followed by the Tukey post-hoc test. * p < 0.05, ** p < 0.01; NS: not significant. Source data are provided as a Source Data file. Full size image We also investigated the subcellular localization of p-Ulk1 746 by immunostaining using this antibody. Consistent with immunoprecipitation-western blotting, a strong p-Ulk1 746 signal appeared in Atg5 KO MEFs upon etoposide treatment (Fig. 1d, f ) in a time-dependent and dose-dependent manner (Supplementary Fig. 3 ). However, these signals were not observed in Atg5 / Ulk1 DKO MEFs and Atg5/Ulk1/Ulk2 triple-knockout ( Atg5 / Ulk1/2 TKO ) MEFs (Supplementary Fig. 4 ) upon etoposide treatment (Fig. 1d, f ). Furthermore, HA-Ulk1 (WT)-expressing, but not HA-Ulk1 (S746A) mutant-expressing Atg5 / Ulk1 DKO MEFs showed p-Ulk1 746 signals after etoposide treatment (Fig. 1e, f ). These findings validate the usefulness of our antibody for immunofluorescence experiments, and again confirmed the etoposide-induced phosphorylation of Ulk1 at Ser 746 . Interestingly, p-Ulk1 746 signals merged almost completely with immunofluorescence signals of the Golgi marker GS28 (Fig. 1d, e ). The Golgi localization of p-Ulk1 746 is reasonable because Golgi membranes are the source of alternative autophagy [5] . Role of Ulk1 Ser 746 phosphorylation in alternative autophagy As we found that etoposide treatment of cells leads to the formation of p-Ulk1 746 on the Golgi and induces alternative autophagy in an Ulk1-dependent manner, we next analyzed the causal relationship between Ulk1 Ser 746 phosphorylation and alternative autophagy. To this end, we analyzed alternative autophagy using red-fluorescent protein (RFP)–green-fluorescent protein (GFP) tandem proteins [18] . Autolysosomes are detected as red puncta because GFP fluorescence, but not RFP fluorescence, becomes weak within acidic lysosomal compartments. Correlative light and electron microscopic (CLEM) analysis confirmed the red puncta as autolysosomes (Fig. 2a , Supplementary Fig. 5 ). As shown in Fig. 2b , red puncta were generated in Atg5 KO MEFs upon etoposide treatment. Furthermore, these red puncta were encircled by immunofluorescence signals of Lamp2 (Fig. 2b ). These findings were confirmed by the fluorescence intensity line profile (Fig. 2b ), indicating the generation of autolysosomes in etoposide-treated Atg5 KO MEFs. Unlike Atg5 KO MEFs, red puncta were not generated in Atg5 / Ulk1 DKO MEFs and Atg5 / Ulk1/2 TKO MEFs after etoposide treatment (Fig. 2c ), and were restored by the expression of HA-Ulk1 (WT) (Fig. 2d ), but not the HA-Ulk1 (S746A) mutant (Fig. 2e ). These results were confirmed by quantitative analysis (Fig. 2f ) and were consistent with the induction of p-Ulk1 746 (Fig. 1f ), indicating the requirement of Ulk1 phosphorylation at Ser 746 for alternative autophagy. Autolysosomes can also be assessed by immunostaining of the lysosomal protein Lamp2, because lysosomal fluorescence increases upon the fusion of lysosomes with autophagic vacuoles. The correspondence of large Lamp2 puncta to autolysosomes was previously shown by CLEM analysis [5] , [8] . Lamp2 immunostaining showed consistent results with the RFP–GFP tandem protein assay (Fig. 2g , Supplementary Fig. 6 ). Note that although etoposide activates both autophagy and apoptosis, we performed all the experiments before apoptosis occurred. Furthermore, similar results were obtained regarding autophagy in cells treated with the pan-caspase inhibitor Q-VD-OPh (Supplementary Fig. 7a, b ), so that the effect of apoptosis could be disregarded. Taken together, Ulk1 phosphorylation at Ser 746 is crucial for etoposide-induced alternative autophagy. Fig. 2: Requirement of Ulk1 phosphorylation at Ser 746 in etoposide-induced alternative autophagy. a CLEM analysis identified red puncta in the autolysosomes of mRFP–GFP-expressing Atg5 KO MEFs. Cells were treated with etoposide (10 µM) for 12 h and observed using fluorescence and electron microscopy. Red puncta were merged with the autophagic vacuoles. Magnified images of the dashed squares are shown in Supplementary Fig. 5 . b – e The indicated MEFs were transiently transfected with the mRFP–GFP plasmid, and after 24 h, cells were treated with etoposide (10 µM) for 15 h, and immunostained with an anti-Lamp2 antibody. Nuclei were counterstained with Hoechst 33342. Representative images are shown. The dashed lines indicate individual cells. Magnified images of the areas within the dashed squares are shown in the insets. Arrowheads indicate mRFP–GFP red puncta (acidic compartments). In b , the fluorescence intensity profile across the white dashed arrows in the inset is shown in the right panel. Note that red puncta were surrounded by Lamp2 signals (arrowheads). f Quantification of cells with mRFP–GFP red puncta. The indicated MEFs were treated with or without 10 µM of etoposide for 15 h. The extent of red puncta was analyzed by the RFP intensity/GFP intensity per cell. Each dot indicates the RFP/GFP ratio in a single cell ( n = 20 cells). Red lines indicate the mean value. Atg5/Ulk1/2 TKO no treatment vs. etoposide: p = 0.9986, Atg5/Ulk1 DKO + HA-Ulk1 (S746A) no treatment vs. etoposide: p = 0.7931. g Quantification of cells with large Lamp2 puncta. The indicated MEFs were treated with or without etoposide (10 µM) for 12 h and immunostained with an anti-Lamp2 antibody. The population of cells with large Lamp2 puncta (≥2 µm) was calculated. ( n ≥ 100 cells in each experiment). Representative images are shown in Supplementary Fig. 6 . Data are shown as the mean ± SD ( n = 3). Atg5/Ulk1/2 TKO , Atg5/Ulk1 DKO + HA-Ulk1 (S746A), no treatment vs. etoposide: p = 0.9797, p = 0.9993, respectively. Comparisons were performed using one-way ANOVA followed by the Tukey post-hoc test. ** p < 0.01; NS: not significant. Source data are provided as a Source Data file. Full size image RIPK3 is essential for the Ulk1 Ser 746 phosphorylation Next, we investigated the kinase responsible for this Ulk1 phosphorylation at Ser 746 . Because the target sequence of Ulk1 at Ser 746 is similar to the sequences of RIPK3 substrates [19] (see section “Discussion”), we focused on RIPK3 [20] . Immunoprecipitation analysis showed the interaction between endogenous RIPK3 and endogenous Ulk1 in untreated conditions (Fig. 3a , lane 7), and an increase in RIPK3 binding from 10 h after etoposide treatment (Fig. 3a , lanes 8 and 9). Such an interaction was not observed in Atg5/RIPK3 double-knockout ( Atg5/RIPK3 DKO ) MEFs (Supplementary Fig. 8a , Fig. 3a , lanes 10–12). Consistently, incubation of lysates from untreated Atg5 KO MEFs, in which Ulk1 746 is not phosphorylated (Fig. 3b , lane 1), with recombinant RIPK3 in phosphorylation buffer resulted in Ulk1 746 phosphorylation (Fig. 3b , lane 2). Furthermore, the phosphorylation of Ulk1 746 was suppressed by the addition of GSK’872, a RIPK3 inhibitor [21] (Fig. 3b , lane 3), indicating that RIPK3 has the potential to phosphorylate Ulk1 at Ser 746 . As expected, etoposide-induced p-Ulk1 746 signals were observed in Atg5 KO MEFs, but not in Atg5/RIPK3 DKO MEFs (Fig. 3c, d , Supplementary Fig. 8b ), which were restored by the exogenous expression of wild-type RIPK3, but not kinase-deficient RIPK3 (Fig. 3c, d ). Consistently, alternative autophagy was observed in Atg5 KO MEFs and wild-type RIPK3-expressing Atg5/RIPK3 DKO MEFs, but not in Atg5/RIPK3 DKO MEFs and kinase-deficient RIPK3-expressing Atg5/RIPK3 DKO MEFs (Fig. 3e, f , Supplementary Fig. 8c, d ). Pharmacological inhibition of RIPK3 by GSK’872 also suppressed etoposide-induced p-Ulk1 746 signals (Fig. 3g, h ) and alternative autophagy (Supplementary Fig. 8e, f ). Consistent with etoposide treatment, camptothecin treatment and ultraviolet C (UVC) exposure, other DNA-damaging treatments also induced the phosphorylation of Ulk1 at Ser 746 in Atg5 KO MEFs, but not in Atg5/RIPK3 DKO MEFs (Supplementary Fig. 9 ). These data indicated that RIPK3 is essential for the genotoxic stress-induced phosphorylation of Ulk1 at Ser 746 and the subsequent induction of alternative autophagy. Fig. 3: Involvement of RIPK3 in the phosphorylation of Ulk1 at Ser 746 and alternative autophagy. a Physical interaction between endogenous Ulk1 and endogenous RIPK3. The indicated MEFs were treated with etoposide (10 µM). Immunoprecipitation was performed with an anti-Ulk1 antibody. Immune complexes and total lysates (2.8% input) were analyzed by western blotting. b In vitro kinase assay of RIPK3 for Ulk1 phosphorylation. Total lysates from untreated Atg5 KO MEFs were incubated with GST-RIPK3 (1 µg) with or without 2 µM of GSK’872 for 1 h. Then, the extent of p-Ulk1 746 was analyzed by immunoprecipitation–western blotting. The arrow indicates the p-Ulk1 746 signal. c – h Requirement of RIPK3 for etoposide-induced phosphorylation of Ulk1 Ser 746 and alternative autophagy. c , d Similar experiments to Fig. 1d were performed using the indicated MEFs. In c , representative images are shown. Arrowheads indicate p-Ulk1 746 signals. In d , the population of cells displaying p-Ulk1 746 signals was calculated ( n ≥ 100 cells). Atg5/RIPK3 DKO , Atg5/RIPK3 DKO + RIPK3 (WT): no treatment vs. etoposide: p = 0.9997, p = 0.0028, respectively. Atg5/RIPK3 DKO vs. Atg5/RIPK3 DKO + RIPK3 (WT): etoposide: p = 0.0099, Atg5/RIPK3 DKO + RIPK3 (WT) vs. Atg5/RIPK3 DKO + RIPK3 (KD): etoposide: p = 0.0041. In e , f , similar experiments to Fig. 2b were performed. Arrowheads indicate mRFP–GFP red puncta. In f , the indicated MEFs were treated with or without 10 µM of etoposide for 15 h. The extent of red puncta was indicated by the RFP/GFP ratio per cell ( n = 20 cells). Red lines indicate the mean value. Atg5/RIPK3 DKO + RIPK3 (KD) no treatment vs. etoposide: p = 0.9376, Atg5/RIPK3 DKO vs. Atg5/RIPK3 DKO + RIPK3 (WT), etoposide: p = 0.0287. g , h Atg5 KO MEFs were treated with etoposide (10 µM) for 12 h with or without GSK’872 (10 µM), and immunostained with anti-p-Ulk1 746 and anti-GS28 antibodies. In g , representative images are shown. p-Ulk1 746 signals were abolished by the addition of GSK’872. In h , the population of cells displaying p-Ulk1 746 signals was calculated ( n ≥ 100 cells). Atg5 KO , Atg5 KO GSK’872: no treatment vs. etoposide: p = 0.0164, p = 0.7853, respectively. Atg5 KO vs. Atg5 KO GSK’872: etoposide: p = 0.0476. In d and h , data are shown as the mean ± SD ( n = 3). Comparisons were performed using one-way ANOVA followed by the Tukey post-hoc test. * p < 0.05, ** p < 0.01. NS: not significant. Source data are provided as a Source Data file. Full size image Etoposide induces both canonical and alternative autophagy. Given that p-Ulk1 746 is crucial for etoposide-induced alternative autophagy, we next investigated whether this phosphorylation is also involved in etoposide-induced canonical autophagy. When MEFs were treated with etoposide, the formation of LC3 puncta was observed in WT MEFs, but not Ulk1/2 DKO MEFs (Fig. 4a ), indicating the loss of canonical autophagy in Ulk1/2 DKO MEFs. The number of cells with LC3 puncta was recovered to a similar level by the expression of the HA-Ulk1 (WT) and the HA-Ulk1 (S746A) mutant (Fig. 4a, b ). Because expression of the HA-Ulk1 (S746A) mutant led to the recovery of canonical autophagy but not alternative autophagy, Ulk1 746 phosphorylation is not involved in etoposide-induced canonical autophagy. Consistent results were obtained when canonical autophagy was assessed by the formation of red puncta in mCherry-GFP-LC3-expressing cells (Supplementary Fig. 10a, b ). Autophagy flux analysis of LC3-II and p62 using bafilomycin A1 confirmed the equivalent induction of canonical autophagy (Fig. 4c ). Therefore, Ulk1 746 phosphorylation is required for etoposide-induced alternative autophagy (Fig. 2 ), but not canonical autophagy. Consistently, despite RIPK3 being essential for etoposide-induced alternative autophagy (Fig. 3 ), canonical autophagy was induced to a similar level in WT MEFs and RIPK3 KO MEFs upon etoposide treatment (Fig. 4d–f , Supplementary Fig. 10c, d ), indicating that RIPK3-dependent Ulk1 phosphorylation at Ser 746 is not involved in etoposide-induced canonical autophagy. Absence of the involvement of Ulk1 746 phosphorylation in canonical autophagy was confirmed because starvation or the addition of rapamycin, both of which strongly induce canonical autophagy but not alternative autophagy, did not generate p-Ulk1 746 signals in WT MEFs (Supplementary Fig. 11a, b ), nor Atg5 KO MEFs (Supplementary Fig. 11c, d ). Furthermore, starvation-induced canonical autophagy was activated to a similar extent in HA-Ulk1 (WT)-expressing and HA-Ulk1 (S746A)-expressing Ulk1/2 DKO MEFs (Supplementary Fig. 12a, b ), as well as in WT MEFs and RIPK3 KO MEFs (Supplementary Fig. 12c, d ). These data indicated the crucial role of RIPK3-dependent generation of p-Ulk1 746 in alternative autophagy, but not in canonical autophagy. Fig. 4: Ulk1 Ser 746 phosphorylation and RIPK3 are not involved in canonical autophagy. a , b The indicated MEFs were treated with or without etoposide (10 µM) for 6 h, and immunostained with an anti-LC3 antibody. Nuclei were counterstained with Hoechst 33342. Representative images of LC3 (red) and Hoechst 33342 (blue) are shown. Magnified images of the areas within the dashed squares are shown in the inset. The population of cells with LC3 puncta b was calculated ( n ≥ 100 cells). Ulk1/2 DKO no treatment vs. etoposide: p = 0.2269. c The indicated MEFs were treated with etoposide (10 µM) for 6 h in the presence or absence of bafilomycin A1 (10 nM), and the expression of each protein was analyzed by western blotting. α-Tubulin was included as a loading control. d – f Similar experiments as a–c were performed using WT and RIPK3 KO MEFs. In e , WT vs. RIPK3 KO etoposide: p = 0.2492. g , h Requirement of RIPK3 for the etoposide-induced generation of p-Ulk1 746 . Similar experiments to Fig. 1d were performed using the indicated MEFs. In g , representative images of p-Ulk1 746 (upper panels) and merged images (lower panels) of p-Ulk1 746 , GS28, and Hoechst 33342 are shown. Arrowheads indicate p-Ulk1 746 signals. In h , the population of cells displaying p-Ulk1 746 signals was calculated ( n ≥ 100 cells). Data are shown as the mean ± SD ( n = 3). Atg5 KO , WT, RIPK3 KO , no treatment vs. etoposide: p = 0.0003, p = 0.0085, p = 0.997, respectively. WT vs. RIPK3 KO etoposide: p = 0.0013. Comparisons were performed using one-way ANOVA followed by the Tukey post-hoc test. ** p < 0.01; NS: not significant. Source data are provided as a Source Data file. Full size image Because RIPK3-dependent p-Ulk1 746 signals were found to be associated with alternative autophagy (Fig. 2 ) but not canonical autophagy (Fig. 4 ), and because we observed these signals in WT MEFs upon etoposide treatment (Fig. 4g, h ), we assumed that alternative autophagy would occur in WT MEFs. Consistent results were obtained when WT thymocytes and RIPK3 KO thymocytes were treated with etoposide (Supplementary Fig. 13a, b ), confirming the crucial role of RIPK3 in the phosphorylation of Ulk1 at Ser 746 upon etoposide treatment. No crosstalk between necroptosis and alternative autophagy In this study, we showed that RIPK3 phosphorylates Ulk1 and thereby induces alternative autophagy upon etoposide treatment. RIPK3 is also known to phosphorylate mixed lineage kinase domain-like (MLKL), and thereby cause membrane rupture, leading to necroptosis when cells are treated with tumor necrosis factor-α (TNF-α), cycloheximide, and the pan-caspase inhibitor zVAD (namely, TCZ [22] ) (Fig. 5a ). Because RIPK3 is used for both alternative autophagy and necroptosis, we tested whether TCZ stimulation induces alternative autophagy, and whether etoposide induces not only apoptosis but also RIPK3/MLKL-mediated necroptosis. The former possibility was denied because TCZ stimulation did not result in p-Ulk1 746 phosphorylation (Fig. 5b , Supplementary Fig. 14a ) and did not induce alternative autophagy, as assessed by Lamp2 puncta formation (Fig. 5c , Supplementary Fig. 14b ). To clarify the latter possibility, we analyzed MLKL phosphorylation and necroptosis induction in etoposide-treated Atg5 KO MEFs. As expected, MLKL activation was not observed (Fig. 5d , lanes 2, 3). Necroptosis was also not induced by etoposide, because cell death was blocked by Q-VD-OPh, but not by Nec-1 and MLKL deletion (Fig. 5e ). Therefore, although RIPK3 was activated by etoposide and TCZ treatment, these stimuli induced alternative autophagy and necroptosis, respectively, without any crosstalk (Fig. 5a ). Fig. 5: Absence of crosstalk between TCZ-induced necroptosis and etoposide-induced alternative autophagy. a (Upper figures) Schematic model of RIPK3-dependent alternative autophagy and TCZ-induced necroptosis. Genotoxic stress induces alternative autophagy via RIPK3-dependent Ulk1 phosphorylation at Ser 746 . TCZ induces necroptosis via RIPK1, RIPK3, and MLKL. (Lower figure) Structure of RIPK3. The kinase and RHIM domains are indicated. Amino acid numbers are shown at the top. T231 and S232 are sites phosphorylated by TCZ treatment. b , c p-Ulk1 746 and alternative autophagy are not induced by TCZ treatment. Atg5 KO MEFs were treated with or without the necroptosis-inducing TCZ solution for 9 h, and then immunostained with anti-p-Ulk1 746 and anti-GS28 antibodies or an anti-Lamp2 antibody. The population of cells displaying p-Ulk1 746 signals b and that of cells containing large Lamp2 puncta (≥2 µm) c was calculated ( n ≥ 100 cells). Data of cells treated with etoposide are shown as a positive control. Representative images are shown in Supplementary Fig. 14 . In b , no treatment vs. etoposide: p = 0.0293, TCZ vs. etoposide: p = 0.0293. In c , TCZ 0 h vs. TCZ 9 h: p = 0.4194, TCZ 0 h vs. TCZ 12 h: p = 0.2938. d MLKL is not activated in etoposide-treated Atg5 KO MEFs. The indicated MEFs were treated with etoposide (10 µM) or TCZ for the indicated times, and phosphorylated MLKL was analyzed by western blotting using an anti-p-MLKL 345 antibody. The p-MLKL signal (arrow) was observed only in TCZ-treated WT MEFs (lane 5). The asterisk indicates a nonspecific band. e Induction of apoptosis, but not necroptosis, by etoposide treatment. The indicated MEFs were treated with etoposide (10 µM) together with Q-VD-OPh (50 µM) or Nec-1 (30 µM) for 16 h, and the population of dead cells was analyzed by the PI uptake assay. WT etoposide vs. WT etoposide/Nec-1: p = 0.864, WT etoposide vs. MLKL KO etoposide: p = 0.1024, WT etoposide/Nec-1 vs. MLKL KO etoposide/Nec-1: p = 0.1791. MLKL KO etoposide vs. MLKL KO etoposide/Nec-1: p = 0.9628. In b , c , and e data are shown as the mean ± SD ( n = 3). Comparisons were performed using one-way ANOVA followed by the Tukey post-hoc test. ** p < 0.01; NS: not significant. Source data are provided as a Source Data file. Full size image We further analyzed the mechanism of RIPK3 activation after etoposide treatment. Upon TCZ treatment, RIPK1 recruits RIPK3 using their RIP homotypic interaction motif (RHIM) domains (Fig. 5a ), which eventually induces RIPK3 homo-oligomerization and generates phospho-RIPK3 231,232 , leading to MLKL activation [23] (Fig. 5a ). In marked contrast, RIPK1 was not required for etoposide-induced p-Ulk1 746 generation, because RIPK1 KO cells normally show p-Ulk1 746 signals (Fig. 6a, b ), unlike RIPK3 KO MEFs (Fig. 3 ). MLKL KO cells also showed normal p-Ulk1 746 signals (Supplementary Fig. 15 ). RIPK3 oligomerization with a subsequent reduction in RIPK3 monomers was induced by TCZ (Fig. 6c , lane 3), but not by etoposide treatment (Fig. 6c , lane 2). Furthermore, although a RHIM domain mutant ( 448 VQIG 451 – 448 AAAA 451 ) did not induce TCZ-induced necroptosis [23] , it still induced equivalent levels of p-Ulk1 746 signals (Fig. 6d, e ) and alternative autophagy (Fig. 6f, g ) in Atg5/RIPK3 DKO MEFs. Deletion mutant analysis supported that kinase domain, but not RHIM domain, was required for RIPK3–Ulk1 interaction (Supplementary Fig. 16 ). Moreover, unlike TCZ treatment, etoposide did not generate phospho-RIPK3 231,232 signals (Fig. 6h, i , lanes 1–3). Taken together, etoposide treatment activates RIPK3 via a completely different mechanism from TCZ treatment. Fig. 6: Different mechanisms of RIPK3 activation by etoposide and TCZ treatment. a , b RIPK1 is not involved in alternative autophagy. RIPK1 KO cells were treated with or without etoposide (10 µM) for 12 h, and immunostained with anti-p-Ulk1 746 and anti-GS28 antibodies. Arrowheads indicate p-Ulk1 746 signals. b The population of cells displaying p-Ulk1 746 signals was calculated ( n ≥ 100 cells). p = 0.025. c Lack of RIPK3 oligomerization by etoposide treatment. The indicated MEFs were treated with or without etoposide or TCZ for 10 h. Cells were then incubated with 2 mM DTBP for 30 min. Nonreduced lysates were subjected to western blotting. Note the increase in oligomer bands and the decrease in the monomer band only by TCZ treatment. d – g No requirement of the RHIM domain in etoposide-induced alternative autophagy. Similar experiments to Figs. 1d and 2b were performed using Flag-RIPK3 (WT)-transfected Atg5/RIPK3 DKO MEFs and Flag-RIPK3 (RHIM mutant)-transfected Atg5/RIPK3 DKO MEFs. Representative images are shown in d . Magnified images are shown in the insets. Arrowheads indicate p-Ulk1 746 signals. In e , the population of cells displaying p-Ulk1 746 signals was calculated ( n ≥ 100 cells). Atg5/RIPK3 DKO + RIPK3 (WT): no treatment vs. etoposide: p = 0.0004, Atg5/RIPK3 DKO + RIPK3 (WT) vs. Atg5/RIPK3 DKO + RIPK3 (RHIM mutant): etoposide: p = 0.0545. Representative images are shown in f . Arrowheads indicate mRFP–GFP red puncta. In g , the extent of red puncta was indicated by the RFP/GFP ratio per cell ( n = 20 cells). Red lines indicate the mean value. Atg5/RIPK3 DKO + RIPK3 (WT) vs. Atg5/RIPK3 DKO + RIPK3 (RHIM mutant) etoposide: p = 0.997. h , i p-RIPK3 231,232 is not induced in etoposide-induced alternative autophagy. The indicated MEFs were treated with etoposide (10 µM) or TCZ for 10 h. In h , cells were immunostained with anti-p-RIPK3 231,232 and anti-GS28 antibodies. In i , the expression of each protein was analyzed by western blotting. The p-RIPK3 231,232 signal (arrow) was observed in TCZ-treated MEFs, but not etoposide-treated MEFs. In b and e , data are shown as the mean ± SD ( n = 3). Comparisons were performed using unpaired two-tailed Student t -tests in b or using one-way ANOVA followed by the Tukey post-hoc test e and g . * p < 0.05; ** p < 0.01; NS: not significant. Source data are provided as a Source Data file. Full size image Requirement of Ulk1 Ser 637 dephosphorylation How does etoposide induce RIPK3-mediated Ulk1 746 phosphorylation? We previously reported that etoposide induced the dephosphorylation of Ulk1 at Ser 637 , a different phosphorylation site, in a manner dependent on p53 and PPM1D [14] . We thus investigated whether Ulk1 637 dephosphorylation is required for Ulk1 746 phosphorylation and alternative autophagy. To this end, we expressed a phosphomimetic (S637D) and a phosphodeficient (S637A) Ulk1 mutants in Atg5/Ulk1 DKO MEFs (Fig. 7a ). The expression of WT Ulk1 and the S637A mutant, but not the S637D mutant, restored the phosphorylation of Ulk1 at Ser 746 (Fig. 7b, c ), as well as alternative autophagy (Fig. 7d , Supplementary Fig. 17 ), despite being expressed at levels similar to those of HA-Ulk1 (Fig. 7a ). This etoposide-induced dephosphorylation at Ser 637 of Ulk1 occurs via p53 and downstream of PPM1D (ref. [14] and Fig. 7e ). Consistent with the results of experiments using Ulk1 mutants of Ser 637 , etoposide-induced phosphorylation of Ulk1 at Ser 746 (Fig. 7f, g ) and alternative autophagy (Fig. 7h, i , Supplementary Fig. 18 ) were observed in Atg5 KO MEFs, but not in Atg5/p53 DKO MEFs and Atg5/PPM1D DKO MEFs. These data indicate that p53/PPM1D-dependent dephosphorylation of Ulk1 at Ser 637 is required for the RIPK3-induced phosphorylation of Ulk1 at Ser 746 and the subsequent induction of alternative autophagy. This notion is supported by the fact that expression of the HA-Ulk1 (S637A) mutant resulted in Ulk1 746 phosphorylation and the induction of alternative autophagy in Atg5/PPM1D DKO MEFs (Supplementary Fig. 19 ). This was further confirmed by the induction of alternative autophagy upon the expression of the HA-Ulk1 (S637A and S746D) mutants (PPM1D-dephosphomimetic and RIPK3-phosphomimetic, respectively) without any stimuli (Supplementary Fig. 20 ). Collectively, the p53–PPM1D axis is required for p53–RIPK3-dependent Ulk1 746 phosphorylation and alternative autophagy. Fig. 7: Requirement of p53/PPM1D-dependent dephosphorylation of Ulk1 at Ser 637 before the phosphorylation of Ulk1 at Ser 746 . a Expression of HA-Ulk1 mutants in Atg5/Ulk1 DKO cells was confirmed by western blotting. b , c The indicated MEFs were treated with or without etoposide (10 µM) for 12 h, and immunostained with anti-p-Ulk1 746 and anti-GS28 antibodies. In b , representative images of p-Ulk1 746 and merged images are shown. Arrowheads indicate p-Ulk1 746 signals. In c , the population of cells displaying p-Ulk1 746 signals was calculated ( n ≥ 100 cells). Atg5/Ulk1 DKO + HA-Ulk1 (S637A) no treatment vs. etoposide: p = 0.0012. d The indicated MEFs were treated with or without etoposide (10 µM) for 12 h, and immunostained with anti-Lamp2 antibody. The population of cells containing large Lamp2 puncta was calculated ( n ≥ 100 cells). Representative images are shown in Supplementary Fig. 17 . Atg5/Ulk1 DKO + HA-Ulk1 (S637A) no treatment vs. etoposide: p = 0.0108. e Effects of p53 and PPM1D in the etoposide-induced modification of Ulk1. The indicated MEFs were treated with etoposide (10 µM) for the indicated times, and the expression of each protein was analyzed by western blotting. f , g Requirement of p53 and PPM1D for the etoposide-induced phosphorylation at Ulk1 Ser 746 . Similar experiments to Fig. 1d were performed. In f , representative images of p-Ulk1 746 and merged images are shown. Arrowheads indicate p-Ulk1 746 signals. In g , the population of cells displaying p-Ulk1 746 signals was calculated ( n ≥ 100 cells). p-Ulk1 746 signals were not observed in Atg5/p53 DKO MEFs and Atg5/PPM1D DKO MEFs. Atg5/PPM1D DKO , no treatment vs. etoposide: p = 0.9933. h , i Requirement of p53 and PPM1D for etoposide-induced alternative autophagy. Similar experiments to Fig. 2b were performed using the indicated MEFs. In h , representative images are shown. Arrowheads indicate mRFP–GFP red puncta. In i , the extent of red puncta was indicated by the RFP/GFP ratio per cell ( n = 20 cells). Red lines indicate the mean value. Atg5/p53 DKO , no treatment vs. etoposide: p = 0.9201, Atg5/PPM1D DKO , no treatment vs. etoposide: p = 0.9987. In c , d , and g data are shown as the mean ± SD ( n = 3). Comparisons were performed using one-way ANOVA followed by the Tukey post-hoc test. ** p < 0.01; NS: not significant. Source data are provided as a Source Data file. Full size image We further elucidated how RIPK3 is activated upon etoposide treatment. Because western blot analysis showed the upregulation of RIPK3 in Atg5 KO MEFs in response to etoposide treatment (Fig. 6i , lanes 2 and 3), we suspected the involvement of p53, a master regulator of genotoxic stress. As expected, RIPK3 upregulation was observed in Atg5 KO cells (Fig. 8a ). However, RIPK3 expression was dramatically suppressed in Atg5/p53 double-knockout ( Atg5/p53 DKO ) MEFs (Fig. 8a ). Very weak expression of RIPK3 was confirmed using different p53 KO MEFs (Supplementary Fig. 21a ) and by the analysis of mRNA levels (Fig. 8b ). Thus, RIPK3 activation upon genotoxic stress was thought to be induced by p53-dependent transcriptional upregulation. The importance of this RIPK3 upregulation was confirmed by the results that the simple expression of RIPK3, but not that of kinase-deficient RIPK3, was sufficient in generating p-Ulk1 746 in HA-Ulk1 (S637A)-expressing Atg5/Ulk1 DKO MEFs (Supplementary Fig. 21b, c ). Neither the phosphorylation of Ulk1 Ser 746 nor the induction of alternative autophagy were observed in Atg5/p53 DKO MEFs was already shown (Fig. 7f–i ). Collectively, upon etoposide treatment, Ulk1 at Ser 637 is dephosphorylated by the p53–PPM1D axis and then phosphorylated by the p53–RIPK3 axis. Thus, p53 plays a dual role in the phosphorylation of Ulk1 at Ser 746 . Fig. 8: Mechanism of Ulk1 746 phosphorylation during etoposide treatment. a , b Crucial role of p53 in RIPK3 activation. The indicated MEFs were treated with etoposide (10 µM) for the indicated times. In a , the expression of each protein was analyzed by western blotting. In b , RIPK3 mRNA and 18S rRNA levels were analyzed using real-time PCR and their ratios were calculated. Values indicate the ratio to “ Atg5 KO time 0”. Data are shown as the mean ± SD ( n = 3). Atg5 KO , no treatment vs. etoposide: p = 0.0029, Atg5 KO vs. Atg5/p53 DKO etoposide: p = 0.0023. c , d RIPK3–Ulk1 interaction occurs in the cytosol. Atg5 KO MEFs were transfected with an expression vector for galactose transferase-fused GFP (GT-GFP); a trans- Golgi marker, and treated with or without etoposide (10 µM). The physical interaction between RIPK3 and Ulk1 was analyzed using Duolink reagents. All Duolink signals were localized in the cytosol. In d , the number of Duolink signals were counted ( n = 50 cells). Red bars indicate mean values. p = 7.4 × 10 −7 . e , f Phosphorylation-dependent translocation of Ulk1 to the Golgi. e The indicated MEFs were transfected with GT-GFP and treated with or without etoposide (10 µM), and assayed with Duolink reagents using anti-Ulk1/anti-GS28 antibodies. In f , the number of Duolink red signals were counted ( n = 50 cells). Red bars indicate mean values. Atg5/Ulk1 DKO + HA-Ulk1 (WT) vs. Atg5/Ulk1 DKO + HA-Ulk1 (S746A), no treatment: p = 0.0137. g Schematic model of the RIPK3-dependent alternative autophagy. Genotoxic stress induces Ulk1 dephosphorylation at Ser 637 in a p53/PPM1D-dependent manner. The dephosphorylated Ulk1 is then phosphorylated at Ser 746 by RIPK3, and translocates to the Golgi, which results in alternative autophagy. h Effect of RIPK3 on the interaction of Ulk1 with Fip200 and Atg13. The indicated MEFs were treated with 10 µM of etoposide (10 µM). Cells were then lysed and immunoprecipitated with an anti-Ulk1 antibody. Immune complexes and total lysates (5.6% input) were analyzed by western blotting. Comparisons were performed using unpaired two-tailed Student t -tests in d or using one-way ANOVA followed by the Tukey post-hoc test in b and f . ** p < 0.01; NS: not significant. Source data are provided as a Source Data file. Full size image We further analyzed where and how RIPK3 phosphorylates Ulk1. To this end, we visualized the interaction between RIPK3 and Ulk1 in Atg5 KO cells using a close proximity (Duolink) assay. As indicated, signals of RIPK3–Ulk1 interaction were increased upon etoposide treatment. Importantly, all signals were localized in the cytosol but not in the Golgi (Fig. 8c, d ), indicating that the RIPK3–Ulk1 interaction occurs in the cytosol. Furthermore, other Duolink assays between HA-Ulk1 and GS28, a pan Golgi marker, showed that etoposide increases the number of HA-Ulk1 (WT)-GS28 signals in Atg5/Ulk1 DKO MEFs (Fig. 8e, f ). The signals were largely decreased when analyzed between HA-Ulk1 (S746A) and GS28 (Fig. 8e, f ), indicating that RIPK3-dependent Ser 746 phosphorylation is important for the translocation of Ulk1 to the Golgi (Fig. 8g ). Fip200 and Atg13 are known as binding partners of Ulk1 in canonical autophagy [2] , [3] . However, their interaction was dramatically decreased in etoposide-treated Atg5 KO MEFs (Fig. 8h , lanes 7–9), and this decrease was not observed, but was rather increased, in Atg5/RIPK3 DKO cells (Fig. 8h , lanes 10–12), indicating that Ulk1 phosphorylation at Ser 746 and Golgi translocation facilitate dissociation of the Ulk1/Fip200/Atg13 complex during alternative autophagy. Consistently, when we analyzed the interaction of HA-Ulk1 (S746D) and HA-Ulk1 (S746A) with Atg13/Fip200 in Atg5/Ulk1 DKO MEFs upon etoposide treatment, we observed a positive interaction for HA-Ulk1 (S746A), but not for HA-Ulk1 (S746D) (Supplementary Fig. 22a ). Furthermore, Fip200 and Atg13 were not localized to the Golgi in etoposide-treated Atg5 KO MEFs (Supplementary Fig. 22b, c ). Therefore, Ulk1 dissociation from the Ulk1/Fip200/Atg13 complex may be important for the recruitment of other target substrates to the Golgi. Taken together, RIPK3 phosphorylates dephospho-Ulk1 637 in the cytosol, and p-Ulk1 746 translocates to the Golgi (Fig. 8g ). Biological roles of etoposide-induced alternative autophagy We finally addressed the biological roles of etoposide-induced alternative autophagy. First, we analyzed the effects of alternative autophagy on apoptosis, because we previously showed that the degradation of Noxa inhibits genotoxic stress-induced apoptosis by canonical autophagy [14] . However, genotoxic stress-induced thymocyte cell death was not altered by RIPK3 (Supplementary Fig. 23a, b ), and Noxa expression levels were also unaffected (Supplementary Fig. 23c ). Similar results were obtained when using splenocytes (Supplementary Fig. 23d, e ). Because RIPK3 deficiency blocks alternative autophagy, these results demonstrate that apoptosis may not be regulated by alternative autophagy, at least in thymocytes and splenocytes. We next focused on Golgi trafficking, because we previously showed that alternative autophagy is induced by the disturbance of Golgi-mediated trafficking for the degradation of undelivered cargos [8] . Thus, we suspected that etoposide also disturbs Golgi trafficking and that alternative autophagy degrades undelivered Golgi cargos. Consistently, genotoxic stress-induced alterations of Golgi morphology has already been reported [24] . To investigate the association between genotoxic stress and Golgi trafficking, we expressed the vesicular stomatitis virus ts045 G protein fused to GFP (VSVG–GFP) in Atg5 KO MEFs [8] , and analyzed their location and degradation (Fig. 9a ). VSVG–GFP was synthesized and remained in the ER at the restrictive temperature (40 °C) (Fig. 9b , image 1). By shifting to the permissive temperature (32 °C), it was transported to the Golgi for 15 min, which was confirmed by its merge with the Golgi marker GS28 (Fig. 9b , image 2), and was delivered to the plasma membrane (PM) in 60 min (Fig. 9b , image 3). However, etoposide treatment suppressed this delivery, because of the low expression of PM-localized VSVG–GFP even at 60 min after the temperature shift (Fig. 9b , image 6). The low expression of PM-localized VSVG–GFP was confirmed using flow cytometry (Fig. 9c ). Interestingly, we observed some VSVG–GFP not only in the Golgi, but also in lysosomes (as assessed by Lamp2 staining), which was substantially increased by the addition of E64d/pepstatin, broad inhibitors of lysosomal proteases (Fig. 9d arrows). Quantitative analysis confirmed the increase in cellular VSVG–GFP levels by E64d/pepstatin (Fig. 9e ). Because E64d/pepstatin inhibits intralysosomal degradation, this indicates that alternative autophagy is utilized for the degradation of untransported VSVG–GFP upon etoposide treatment. In contrast to Atg5 KO MEFs, in Atg5/RIPK3 DKO MEFs, VSVG–GFP was observed not only on the Golgi but also in the cytoplasmic punctate structures at 60 min (Fig. 9b , compare images 6 and 12). A higher expression level of VSVG–GFP in Atg5/RIPK3 DKO MEFs than that in Atg5 KO MEFs was quantitatively confirmed (Fig. 9e ). Furthermore, E64d/pepstatin did not show any effects on VSVG–GFP localization (Fig. 9d ) and expression levels (Fig. 9e ), and colocalization of VSVG–GFP and Lamp2 was only rarely observed in Atg5/RIPK3 DKO MEFs, which indicates that VSVG–GFP was not engulfed by autolysosomes. Therefore, RIPK3-dependent alternative autophagy is thought to play a role in eliminating superfluous undelivered proteins from the Golgi in etoposide-treated MEFs. Consistent results were obtained when cells were treated with camptothesin (Supplementary Fig. 24 ). We also performed the VSVG–GFP trafficking assay using Atg5/Ulk1 DKO MEF derivatives and found that HA-Ulk1 (WT)-expressin g Atg5/Ulk1 DKO MEFs and HA-Ulk1 (S746A)-expressing Atg5/Ulk1 DKO MEFs showed similar results to Atg5 KO MEFs and Atg5/RIPK3 DKO MEFs, respectively (Supplementary Fig. 25 ), indicating that p-Ulk1 746 -dependent alternative autophagy plays a role in eliminating undelivered VSVG–GFP in etoposide-treated MEFs. Fig. 9: Effect of RIPK3 on the degradation of undelivered VSVG upon etoposide treatment. a Schematic diagram of the experiment. The VSVG–GFP was expressed in Atg5 KO MEFs and Atg5/RIPK3 DKO MEFs, and the cells were treated with or without etoposide (10 µM) at the restrictive temperature (40 °C) for 12 h. Cells were then shifted to the permissive temperature (32 °C), and fixed at the indicate times. Golgi was counterstained with an anti-GS28 antibody. b Representative images are shown. At 0, 15, and 60 min after the temperature shift, the location of VSVG–GFP and Golgi were analyzed. c Reduction of PM-localized VSVG–GFP upon etoposide treatment. VSVG–GFP-expressing Atg5 KO MEFs were or were not treated with etoposide, and at 60 min after the temperature shift, cells were stained with an anti-VSVG antibody for 30 min at 4 °C followed by the addition of an Alexa Fluor 633-conjugated secondary antibody for 30 min at 4 °C. After washing the cells, the amount of PM-localized VSVG–GFP was measured using flow cytometry. d , e VSVG–GFP-expressing Atg5 KO MEFs and Atg5/RIPK3 DKO MEFs were treated with etoposide (10 µM) in the presence of E64d/pepstatin. At 60 min after the temperature shift, cells were immunostained with an anti-Lamp2 antibody. In d , representative images are shown. Arrowheads indicate autolysosomes containing VSVG–GFP. A magnified image of the areas within the dashed squares is shown in the insets. In e , the amount of total VSVG–GFP (the level of fluorescence intensity in each cell) was measured using Image J ( n = 30 cells in each experiment). Red bars indicate mean values. Atg5 KO Etoposide vs. Etoposide with E64d/pepstatin: p = 0.0043, Atg5/RIPK3 DKO Etoposide vs. Etoposide with E64d/pepstatin: p = 0.6495. Comparisons were performed using one-way ANOVA followed by the Tukey post-hoc test. ** p < 0.01; NS: not significant. Source data are provided as a Source Data file. Full size image Because VSVG–GFP is an artificial substrate used to monitor Golgi trafficking, we further analyzed integrin alpha5 as an example of an endogenous cargo that is trafficked by the Golgi. Integrin alpha5 mostly localized to focal adhesions in Atg5 KO MEFs (Fig. 10a ). Upon the addition of etoposide and E64d/pepstatin, we observed multiple integrin alpha5 puncta encircled by Lamp1 (Fig. 10a , image 9), which are thought to be autolysosomes. In contrast, in Atg5/RIPK3 DKO MEFs, etoposide generated unusual cytoplasmic integrin alpha5 puncta (Fig. 10a , image 13), which should be the undelivered and undegraded integrin alpha5. E64d/pepstatin did not show any effects on this integrin alpha5 localization (Fig. 10a , image 16) and expression (Fig. 10b ). Consistently, merged puncta of integrin alpha5 and Lamp1 were only rarely observed in Atg5/RIPK3 DKO MEFs (Fig. 10a , image 18). HA-Ulk1 (WT)-expressin g and HA-Ulk1 (S746A)-expressing Atg5/Ulk1 DKO showed similar results with Atg5 KO MEFs and Atg5/RIPK3 DKO MEFs, respectively (Supplementary Fig. 26 ). Taken together, RIPK3/p-Ulk1 746 -dependent alternative autophagy plays a role in eliminating undelivered Golgi cargos upon genotoxic stress. Fig. 10: Requirement of RIPK3 for undelivered integrin α5 degradation upon etoposide treatment. The Atg5 KO MEFs and Atg5/RIPK3 DKO MEFs were treated with or without etoposide (10 µM) in the presence of E64d/pepstatin for 12 h. Cells were immunostained with anti-Lamp1 and anti-integrin α5 antibodies. In a , representative images are shown. Arrows and arrowheads indicate unusual cytoplasmic integrin alpha5 puncta and integrin α5 engulfed in autolysosomes, respectively. Magnified images of the areas within the dashed squares are shown in the insets. Note that etoposide generated unusual cytoplasmic integrin alpha5 puncta in Atg5/RIPK3 DKO MEFs. In b , the amount of total integrin α5 (the level of fluorescence intensity per cell) was measured ( n = 30 cells in each experiment). Red bars indicate mean values. Atg5 KO vs. Atg5/RIPK3 DKO Etoposide: p = 0.0093, Atg5/RIPK3 DKO Etoposide vs. Etoposide with E64d/pepstatin: p = 0.744. Comparisons were performed using one-way ANOVA followed by the Tukey post-hoc test. ** p < 0.01; NS: not significant. Source data are provided as a Source Data file. Full size image Both canonical and alternative autophagy are initiated by Ulk1 activation, but the mechanism as to how Ulk1 activates these different pathways has remained unknown. We here demonstrated that the phosphorylation of Ulk1 at Ser 746 is the key difference between the two autophagy pathways, because the extent of Ulk1 746 phosphorylation determines the induction of alternative autophagy but not canonical autophagy. Therefore, the induction of p-Ulk1 746 should be a good marker of alternative autophagy. Ulk1 is usually located throughout the cytosol, and upon genotoxic stress, a proportion of Ulk1 is phosphorylated at Ser 746 by RIPK3 in the cytosol. How does p-Ulk1 746 localize on the Golgi? First, genotoxic stress dephosphorylates Ulk1 at Ser 637 in a manner dependent on p53 and PPM1D. This dephosphorylation is important for both canonical and alternative autophagy. Next, p53-upregulated RIPK3 associates with and phosphorylates Ulk1 at Ser 746 in the cytosol, and subsequently p-Ulk1 746 translocates to the Golgi. It is thought that Ser 637 dephosphorylation is required for the structural alteration of Ulk1, which is required for the phosphorylation on Ulk1 746 . Phosphorylated Ulk1 746 should dissociate from Fip200/Atg13, a complex required for canonical autophagy, and instead, it translocates to the Golgi and interacts with and phosphorylates yet unidentified substrates that are localized on the Golgi, to induce alternative autophagy. We here identified RIPK3 as the upstream kinase of Ulk1 during etoposide-induced alternative autophagy. RIPK3 is also known as the upstream kinase of MLKL during TCZ-induced necroptosis [22] , [23] . For MLKL activation, RIPK3 recruitment by RIPK1, RHIM domain-mediated RIPK3 oligomerization, and phosphorylation of RIPK3 on Thr 231 /Ser 232 are required. In contrast, for etoposide-induced Ulk1 phosphorylation, RIPK3 activation occurs independently of RIPK1, RIPK3 oligomerization, and p-RIPK3 231,232 generation. Instead, it occurs via the p53-dependent transcriptional upregulation. Then, the upregulated RIPK3 phosphorylates Ulk1 in the cytosol. Because there are several other RIPK3 target molecules, such as metabolic enzymes [25] (glycogen phosphorylase L, glutamate-ammonia ligase, and glutamate dehydrogenase 1) in the cytosol, these substrates might also be activated and play a role in various cellular events. The major phosphorylation consensus motifs of RIPK3 are phospho-Thr/phospho-Ser/Met, phospho-Ser/Pro, and phospho-Ser/X/Pro [19] , [22] , [26] . The position of Ulk1 746 (phospho-Ser/Ser/Pro) fits with this consensus motif, whereas Ulk2 does not have any Ser/Ser/Pro or Ser/Pro sequences in the local vicinity of the alignment locations (Supplementary Fig. 1e ). Therefore, RIPK3 may only target Ulk1, but not Ulk2, upon genotoxic stress. Because Atg5/Ulk1 DKO MEFs and Atg5/RIPK 3 DKO MEFs were largely resistant to genotoxic stress-induced alternative autophagy, the contribution of Ulk2 to genotoxic stress-induced alternative autophagy appears to be small. Of course, we do not deny the possibility that Ulk2 plays a role in alternative autophagy in other contexts. Taken together, we here identified a phosphorylation site (Ser 746 ) of Ulk1, which is phosphorylated upon genotoxic stress in a RIPK3-dependent manner. p-Ulk1 746 localizes solely to the Golgi, and is essential for alternative autophagy, but not canonical autophagy. Mice RIPK3 KO mice [20] and PPM1D KO mice [27] were kind gifts from Genentech Co. and Professor L.A. Donehower, respectively. Mice were bred in a 12 h light/12 h dark cycle at ~23 °C and 40% relative humidity at the Laboratory for Recombinant Animals of Tokyo Medical and Dental University, Tokyo, Japan. The Tokyo Medical and Dental University Ethics Committee for Animal Experiments approved all experiments in this study, and all experiments were performed according to their regulations. 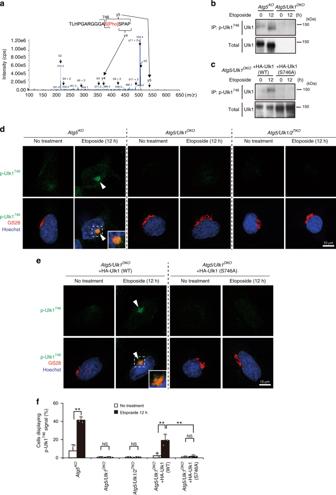Fig. 1: Phosphorylation of Ulk1 at Ser746and its Golgi localization upon etoposide treatment. aIdentification of an Ulk1 phosphorylation site. Ulk1 was immunoprecipitated with the anti-Ulk1 antibody from etoposide-treatedAtg5KOMEFs and subjected to trypsin digestion. The tryptic digests were analyzed by LC–MS/MS. This mass spectrum yielded a fragment ion spectrum displaying three C-terminal fragment ions (y-type) and seven N-terminal fragment ions (b-type). The result that y5-y4 is about 167 Da, which is equivalent to a phosphoserine, and database searching identified this peptide as TLHPGARGGGAS[Pho]SPAP, the partial sequence (amino acids 735–750) of the Ulk1 protein.b,cPhosphorylation of Ulk1 at Ser746by etoposide treatment. The indicated MEFs were treated with 10 µM of etoposide for the indicated times, lysed, and immunoprecipitated with an anti-p-Ulk1746antibody. Immune complexes and total lysates (2.8% input) were analyzed by western blotting using an anti-Ulk1 antibody.d,eInduction of the Golgi localization of p-Ulk1746by etoposide treatment. The indicated MEFs were treated with or without 10 µM of etoposide for 12 h, and immunostained with anti-p-Ulk1746and anti-GS28 antibodies. Nuclei were counterstained with Hoechst 33342 (50 ng mL−1). Representative images of p-Ulk1746(green; upper panels) and merged images (lower panels) of p-Ulk1746(green), GS28 (red), and Hoechst 33342 (blue) are shown. Magnified images of the areas within the dashed squares are shown in the inset. Arrowheads indicate p-Ulk1746signals.fQuantification of cells displaying p-Ulk1746signals. The indicated MEFs were treated with 10 µM of etoposide for the indicated times, and immunostained with an anti-p-Ulk1746antibody. The population of cells with p-Ulk1746signals was calculated (n≥ 100 cells in each experiment). Data are shown as the mean ± SD (n= 3).Atg5/Ulk1DKO+ HA-Ulk1 (WT) no treatment vs. etoposide:p= 0.0002. Other exactpvalues cannot be described since the value is too large (p> 0.9999) or small (p< 0.0001). Comparisons were performed using one-way ANOVA followed by the Tukey post-hoc test. *p< 0.05, **p< 0.01; NS: not significant. Source data are provided as a Source Data file. Antibodies and chemicals The antibodies used are listed in Supplementary Table 1 . Etoposide, bafilomycin A1, cycloheximide, Q-VD-OPh, camptothecin, and GSK’872 were obtained from Sigma-Aldrich, Adipogen, Wako, R&D systems, Wako, and Calbiochem, respectively. All other chemicals were purchased from Nacalai Tesque. Plasmid construction The HA-tagged mouse Ulk1 plasmid was a kind gift from Professor Muramatsu (Tokyo Medical and Dental University). The introduction of point mutations into mouse Ulk1 was performed using PCR with Pfu Turbo (Agilent Technologies). The introduction of deletion mutations into mouse RIPK3 was performed using PCR with PrimeSTAR GXL (Takara). An expression vector for the galactose transferase plasmid [28] was a kind gift from Animal Resource Development & Genetic Engineering, Center for Life Science Technologies, RIKEN. All constructs were confirmed by sequence analysis. 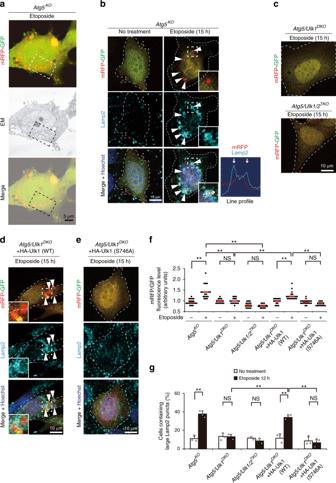Fig. 2: Requirement of Ulk1 phosphorylation at Ser746in etoposide-induced alternative autophagy. aCLEM analysis identified red puncta in the autolysosomes of mRFP–GFP-expressingAtg5KOMEFs. Cells were treated with etoposide (10 µM) for 12 h and observed using fluorescence and electron microscopy. Red puncta were merged with the autophagic vacuoles. Magnified images of the dashed squares are shown in Supplementary Fig.5.b–eThe indicated MEFs were transiently transfected with the mRFP–GFP plasmid, and after 24 h, cells were treated with etoposide (10 µM) for 15 h, and immunostained with an anti-Lamp2 antibody. Nuclei were counterstained with Hoechst 33342. Representative images are shown. The dashed lines indicate individual cells. Magnified images of the areas within the dashed squares are shown in the insets. Arrowheads indicate mRFP–GFP red puncta (acidic compartments). Inb, the fluorescence intensity profile across the white dashed arrows in the inset is shown in the right panel. Note that red puncta were surrounded by Lamp2 signals (arrowheads).fQuantification of cells with mRFP–GFP red puncta. The indicated MEFs were treated with or without 10 µM of etoposide for 15 h. The extent of red puncta was analyzed by the RFP intensity/GFP intensity per cell. Each dot indicates the RFP/GFP ratio in a single cell (n= 20 cells). Red lines indicate the mean value.Atg5/Ulk1/2TKOno treatment vs. etoposide:p= 0.9986,Atg5/Ulk1DKO+ HA-Ulk1 (S746A) no treatment vs. etoposide:p= 0.7931.gQuantification of cells with large Lamp2 puncta. The indicated MEFs were treated with or without etoposide (10 µM) for 12 h and immunostained with an anti-Lamp2 antibody. The population of cells with large Lamp2 puncta (≥2 µm) was calculated. (n≥ 100 cells in each experiment). Representative images are shown in Supplementary Fig.6. Data are shown as the mean ± SD (n= 3).Atg5/Ulk1/2TKO,Atg5/Ulk1DKO+ HA-Ulk1 (S746A), no treatment vs. etoposide:p= 0.9797,p= 0.9993, respectively. Comparisons were performed using one-way ANOVA followed by the Tukey post-hoc test. **p< 0.01; NS: not significant. Source data are provided as a Source Data file. The primers used are listed in Supplementary Table 2 . Cell culture and DNA transfection MEFs were generated from WT, Atg5 KO , Atg5/Ulk1 DKO , RIPK3 KO , Atg5/p53 DKO , Atg5/PPM1D DKO , and Mlkl KO embryos on embryonic day 14.5 by immortalization with the SV40 T antigen. To generate MEFs stably expressing RIPK3, HA-Ulk1, and its mutants, each plasmid was transfected into MEFs (1 × 10 6 ) using the Amaxa electroporation system (Lonza) and selected using hygromycin B (Invivogen). For transient DNA transfection, cells were transfected with the Neon electroporation system (Invitrogen) according to the manufacturer’s instructions. Atg5/RIPK3 DKO MEFs were generated from RIPK3 KO MEFs by the CRISPR/Cas9 system [29] . Briefly, a 20-bp mouse Atg5-targeting sequence (GAGAGTCAGCTATTTGACGT) was synthesized (Eurofins) and inserted into the px330 plasmid [8] (Addgene). This plasmid was also transfected into Ulk1/2 DKO MEFs. Then, a single colony of Atg5/Ulk1/2 TKO and Atg5/RIPK3 DKO MEFs was obtained, and Atg5 deficiency was confirmed by western blotting against Atg5 and LC3. WT and RIPK3 KO primary thymocytes were harvested from the respective mice at 5–6 weeks of age. MEFs and thymocytes were cultured in Dulbecco’s modified Eagle’s medium supplemented with 2 mM l -glutamine, 1 mM sodium pyruvate, 0.1 mM nonessential amino acids, 10 mM HEPES/Na + (pH 7.4), 0.05 mM 2-mercaptoethanol, 100 U/mL penicillin, 100 μg/mL streptomycin, and 10% fetal bovine serum [10] . 293T cells were transfected with Lipofectamine 2000 (Thermo Fisher Scientific) according to the manufacturer’s instructions. Mass-spectrometry analysis Mass-spectrometry analysis was performed as follows [30] . Anti-Ulk1 immunoprecipitates from non-treated or etoposide-treated Atg5 KO MEFs were separated by 5–20% SDS–PAGE, and stained by silver staining (SilverQuest staining kit, Invitrogen). The gel bands around 150 kDa were cut out, treated with dithiothreitol (10 mM), dissolved in ammonium hydrogen carbonate (100 mM), and treated with iodoacetamide (40 mM). After the gels were dried, 20 µL of 0.05 pmol L −1 trypsin solution was applied to each gel piece and incubated for 14 h at 37 °C to digest the proteins. Digested peptides were extracted with 50% trifluoroacetic acid (TFA), followed by 80% TFA. The purified peptide samples were injected onto a reversed-phase C18 column (HiQ sil C18W-3P, 3 mm, 120 Å; KYA TECH Co.) and separated by nanoflow liquid chromatography (300 nL min −1 ) on a nano LC Dina-A system (KYA TECH Co.) with a Q-TRAP 5500 mass spectrometer (AB SCIEX). Immunoblot analysis Cells were lysed in cell lysis buffer containing 20 mM HEPES (pH 7.5), 100 mM NaCl, 1.5 mM MgCl 2 , 1 mM EGTA, 10 mM Na 2 P 2 O 7 , 10% glycerol, 1% NP-40, 1 mM dithiothreitol, 1 mM Na 3 VO 4 , and 1% protease inhibitor cocktail. After vortexing for 15 s, insoluble material was removed by centrifugation. Supernatants were loaded onto 5–20%, 15%, or 8% SDS–polyacrylamide gels. After electrophoresis, the proteins were blotted onto PVDF membranes. The membranes were blocked with 5% skim milk in TBS containing 0.05% Tween-20 (TBS-T) and incubated with a primary antibody overnight at 4 °C. After washing with TBS-T, the membranes were incubated with a horseradish peroxidase-labeled secondary antibody and visualized with Chemi-Lumi One Super reagent. All experiments were conducted at least in duplicate. Immunoprecipitation Untreated and etoposide-treated MEFs were harvested and lysed with cell lysis buffer. Immunoprecipitation was performed using an indicated antibody in the presence of protein-G Sepharose (GE Healthcare) for 2 h at 4 °C. The beads were then washed three times with PBS. In experiment using Flag-RIPK3 deletion mutants in HEK293T cells, the beads were washed two times with PBS. Proteins were released from the beads by heating at 100 °C for 3 min in 2 × Laemmli sample buffer. Immunoblotting was performed as described above, except that the EasyBlot anti-rabbit IgG kit (GeneTex) was used to avoid the detection of non-specific IgG bands. Kinase assay Cells were lysed in cell lysis buffer. After vortexing for 15 s, insoluble material was removed by centrifugation. Supernatants were treated with or without 1 µg of GST-RIPK3 together with or without 2 µM of the RIPK3 inhibitor GSK’872, for 1 h at 30 °C, followed by immunoprecipitation with an anti-phospho-Ulk1 746 antibody. The levels of phosph-Ulk1 746 were analyzed by immunoblotting using an anti-Ulk1 antibody and the EasyBlot anti-rabbit IgG kit. Phosphatase assay Cells were lysed in cell lysis buffer containing 20 mM HEPES (pH 7.5), 100 mM NaCl, 1.5 mM MgCl 2 , 1 mM EGTA, 10% glycerol, 1% NP-40, 1 mM dithiothreitol, and 1% protease inhibitor cocktail. After vortexing for 15 s, insoluble material was removed by centrifugation. Supernatants were treated with or without 4000 U of lambda protein phosphatase (λPPase) for 1 h at 30 °C, followed by immunoprecipitation with an anti-phospho-Ulk1 746 antibody. The levels of phosph-Ulk1 746 were analyzed by immunoblotting using an anti-Ulk1 antibody and the EasyBlot anti-rabbit IgG kit. Immunofluorescence analysis Cells were fixed in 4% paraformaldehyde containing 8 mM EGTA for 10 min and then permeabilized using 50 µg mL −1 digitonin for 5 min. Cells were then stained with the indicated primary antibodies for 1 h at room temperature. After washing, the cells were stained with secondary antibodies and Hoechst 33342, mounted in Prolong Gold Antifade reagent, and observed using a fluorescence microscope (IX71, Olympus) and a laser-scanning confocal microscope (LSM710, Zeiss). For staining with the anti-Ser 746 Ulk1 antibody, cells were fixed in 4% paraformaldehyde containing 8 mM EGTA for 5 min and then permeabilized using 20 µg mL −1 digitonin for 2 min on ice to avoid nonspecific nuclear staining. Thymocytes were fixed in 4% paraformaldehyde containing 8 mM EGTA for 5 min, pelleted onto slides using a Cytospin3 centrifuge (Shandon), and permeabilized using 20 µg mL −1 digitonin for 2 min on ice. Cells were then stained as described above. 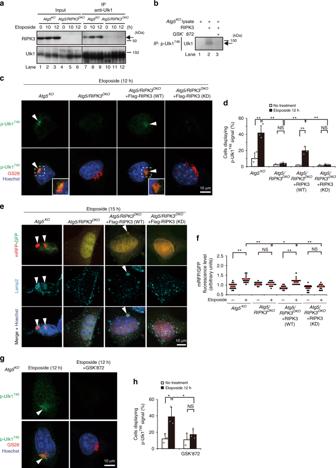Fig. 3: Involvement of RIPK3 in the phosphorylation of Ulk1 at Ser746and alternative autophagy. aPhysical interaction between endogenous Ulk1 and endogenous RIPK3. The indicated MEFs were treated with etoposide (10 µM). Immunoprecipitation was performed with an anti-Ulk1 antibody. Immune complexes and total lysates (2.8% input) were analyzed by western blotting.bIn vitro kinase assay of RIPK3 for Ulk1 phosphorylation. Total lysates from untreatedAtg5KOMEFs were incubated with GST-RIPK3 (1 µg) with or without 2 µM of GSK’872 for 1 h. Then, the extent of p-Ulk1746was analyzed by immunoprecipitation–western blotting. The arrow indicates the p-Ulk1746signal.c–hRequirement of RIPK3 for etoposide-induced phosphorylation of Ulk1 Ser746and alternative autophagy.c,dSimilar experiments to Fig.1dwere performed using the indicated MEFs. Inc, representative images are shown. Arrowheads indicate p-Ulk1746signals. Ind, the population of cells displaying p-Ulk1746signals was calculated (n≥ 100 cells).Atg5/RIPK3DKO,Atg5/RIPK3DKO+ RIPK3 (WT): no treatment vs. etoposide:p= 0.9997,p= 0.0028, respectively.Atg5/RIPK3DKOvs.Atg5/RIPK3DKO+ RIPK3 (WT): etoposide:p= 0.0099,Atg5/RIPK3DKO+ RIPK3 (WT) vs.Atg5/RIPK3DKO+ RIPK3 (KD): etoposide:p= 0.0041. Ine,f, similar experiments to Fig.2bwere performed. Arrowheads indicate mRFP–GFP red puncta. Inf, the indicated MEFs were treated with or without 10 µM of etoposide for 15 h. The extent of red puncta was indicated by the RFP/GFP ratio per cell (n= 20 cells). Red lines indicate the mean value.Atg5/RIPK3DKO+ RIPK3 (KD) no treatment vs. etoposide:p= 0.9376,Atg5/RIPK3DKOvs.Atg5/RIPK3DKO+ RIPK3 (WT), etoposide:p= 0.0287.g,hAtg5KOMEFs were treated with etoposide (10 µM) for 12 h with or without GSK’872 (10 µM), and immunostained with anti-p-Ulk1746and anti-GS28 antibodies. Ing, representative images are shown. p-Ulk1746signals were abolished by the addition of GSK’872. Inh, the population of cells displaying p-Ulk1746signals was calculated (n≥ 100 cells).Atg5KO,Atg5KOGSK’872: no treatment vs. etoposide:p= 0.0164,p= 0.7853, respectively.Atg5KOvs.Atg5KOGSK’872: etoposide:p= 0.0476. Indandh, data are shown as the mean ± SD (n= 3). Comparisons were performed using one-way ANOVA followed by the Tukey post-hoc test. *p< 0.05, **p< 0.01. NS: not significant. Source data are provided as a Source Data file. Data analysis was performed using Zen software 2012 (Zeiss), Adobe photoshop CS5.1, and Illustrator CS5.1. Quantitation of alternative autophagy The extent of alternative autophagy was analyzed by the mRFP–GFP assay and Lamp2 swelling assay. In the experiments using mRFP–GFP, autolysosomes were visualized as red puncta, because GFP fluorescence, but not RFP fluorescence, is decreased in acidic compartments. Therefore, the cellular RFP/GFP fluorescence ratio is increased in autophagy-inducing cells. RFP and GFP images were acquired using Zen software, and analyzed cellular fluorescence intensity (intensity × area per cell) using Image J software. Then, the cellular RFP/GFP level of each cell was obtained. Levels of alternate autophagy were also quantified using the Lamp2 staining assay. As our previous study demonstrated that large Lamp2 puncta (≥2 µm) were identical to autophagic vacuoles [5] , and there were very few such big Lamp2 puncta in non-autophagic cells, cells with more than one large LAMP2 (≥2 µm) punctum was regarded as an autophagic cell, and cells were analyzed using Zen software (Zeiss). Images of Lamp2-stained cells were acquired and the number of cells with large Lamp2 puncta were calculated. Correlative light and electron microscopy To merge photographs from confocal fluorescence microscopy and EM, samples were quick frozen and transferred to 0.00001% OsO 4 and 0.01% glutaraldehyde in acetone (80 °C for 24 h, −30 °C for 6 h, −15 °C for 1 h, and 37 °C for 30 min), and washed with acetone. After replacing the acetone to PBS(−), the samples were visualized by confocal microscopy. Samples were then fixed in Karnovsky solution (1.5% paraformaldehyde and 3% glutaraldehyde in phosphate buffer) for 15 min at room temperature and 1% OsO 4 at 4 °C for 5 min. After dehydration, the samples were embedded in Epon, and thin sections were observed with a JEM 1010 electron microscope at 80 kV. UVC irradiation After replacing the medium with PBS, cells were exposed to 30 J m −2 of UVC light in a UV crosslinker CX-2000 equipped with a UV-lamp. After irradiation, PBS was aspirated and replaced with the culture medium. After cells were incubated for 1 and 3 h, cell were fixed and stained as described above. Duolink in situ proximity ligation assay Cells were fixed in 4% paraformaldehyde containing 8 mM EGTA for 10 min and then permeabilized using 50 µg mL −1 digitonin for 5 min. Cells were then stained with the indicated primary antibodies overnight at 4 °C. After washing, the cells were assayed with Duolink in situ reagents according to the manufacturer’s instructions, and mounted in Prolong Gold Antifade reagent with DAPI (Thermo Fisher Scientific) and a laser-scanning confocal microscope (LSM710, Zeiss). Data analysis was performed using Zen and Image J software. Cell viability assay Cells were stained with propidium iodide (PI) and cell viability was detected by flow cytometry (BD; FACS Canto II). 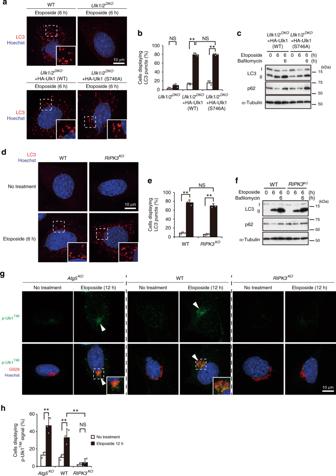Fig. 4: Ulk1 Ser746phosphorylation and RIPK3 are not involved in canonical autophagy. a,bThe indicated MEFs were treated with or without etoposide (10 µM) for 6 h, and immunostained with an anti-LC3 antibody. Nuclei were counterstained with Hoechst 33342. Representative images of LC3 (red) and Hoechst 33342 (blue) are shown. Magnified images of the areas within the dashed squares are shown in the inset. The population of cells with LC3 punctabwas calculated (n≥ 100 cells).Ulk1/2DKOno treatment vs. etoposide:p= 0.2269.cThe indicated MEFs were treated with etoposide (10 µM) for 6 h in the presence or absence of bafilomycin A1 (10 nM), and the expression of each protein was analyzed by western blotting. α-Tubulin was included as a loading control.d–fSimilar experiments asa–cwere performed using WT andRIPK3KOMEFs. Ine, WT vs.RIPK3KOetoposide:p= 0.2492.g,hRequirement of RIPK3 for the etoposide-induced generation of p-Ulk1746. Similar experiments to Fig.1dwere performed using the indicated MEFs. Ing, representative images of p-Ulk1746(upper panels) and merged images (lower panels) of p-Ulk1746, GS28, and Hoechst 33342 are shown. Arrowheads indicate p-Ulk1746signals. Inh, the population of cells displaying p-Ulk1746signals was calculated (n≥ 100 cells). Data are shown as the mean ± SD (n= 3).Atg5KO, WT,RIPK3KO, no treatment vs. etoposide:p= 0.0003,p= 0.0085,p= 0.997, respectively. WT vs.RIPK3KOetoposide:p= 0.0013. Comparisons were performed using one-way ANOVA followed by the Tukey post-hoc test. **p< 0.01; NS: not significant. Source data are provided as a Source Data file. Cell populations were separated from cellular debris using FSC/SSC (Supplementary Fig. 27 ). Data analysis was performed using BD FACSDiva and FlowJo software. Real-time PCR Total RNA was extracted using the Qiagen RNeasy Mini kit. The synthesis of first-strand cDNA and real-time PCR was performed in the CFX96 Real-Time system by using the iTaq universal SYBR green one-step kit (Bio-Rad). Data were collected by CFX manager 3.1 (Bio-Rad). RIPK3 and 18S rRNA primers are listed in Supplementary Table 2 . Expression was normalized using 18S rRNA as an internal control. VSVG and integrin alpha5 trafficking MEFs were transfected with VSVG–GFP and plated, and then treated with or without etoposide (10 µM), E64d (10 µg mL −1 ), and pepstatin (10 µg mL −1 ) at the restrictive temperature for VSVG–GFP (40 °C) for 12 h. Cells were then shifted to the permissive temperature (32 °C), and fixed at the indicated times. Golgi and lysosomes were counterstained with an anti-GS28 and anti-Lamp2 antibody, respectively. 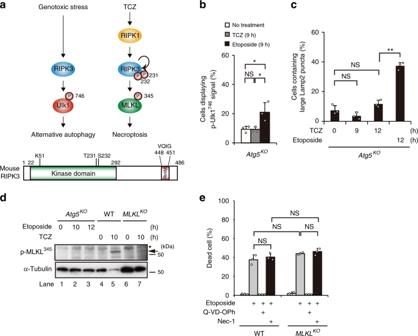Fig. 5: Absence of crosstalk between TCZ-induced necroptosis and etoposide-induced alternative autophagy. a(Upper figures) Schematic model of RIPK3-dependent alternative autophagy and TCZ-induced necroptosis. Genotoxic stress induces alternative autophagy via RIPK3-dependent Ulk1 phosphorylation at Ser746. TCZ induces necroptosis via RIPK1, RIPK3, and MLKL. (Lower figure) Structure of RIPK3. The kinase and RHIM domains are indicated. Amino acid numbers are shown at the top. T231 and S232 are sites phosphorylated by TCZ treatment.b,cp-Ulk1746and alternative autophagy are not induced by TCZ treatment.Atg5KOMEFs were treated with or without the necroptosis-inducing TCZ solution for 9 h, and then immunostained with anti-p-Ulk1746and anti-GS28 antibodies or an anti-Lamp2 antibody. The population of cells displaying p-Ulk1746signalsband that of cells containing large Lamp2 puncta (≥2 µm)cwas calculated (n≥ 100 cells). Data of cells treated with etoposide are shown as a positive control. Representative images are shown in Supplementary Fig.14. Inb, no treatment vs. etoposide:p= 0.0293, TCZ vs. etoposide:p= 0.0293. Inc, TCZ 0 h vs. TCZ 9 h:p= 0.4194, TCZ 0 h vs. TCZ 12 h:p= 0.2938.dMLKL is not activated in etoposide-treatedAtg5KOMEFs. The indicated MEFs were treated with etoposide (10 µM) or TCZ for the indicated times, and phosphorylated MLKL was analyzed by western blotting using an anti-p-MLKL345antibody. The p-MLKL signal (arrow) was observed only in TCZ-treated WT MEFs (lane 5). The asterisk indicates a nonspecific band.eInduction of apoptosis, but not necroptosis, by etoposide treatment. The indicated MEFs were treated with etoposide (10 µM) together with Q-VD-OPh (50 µM) or Nec-1 (30 µM) for 16 h, and the population of dead cells was analyzed by the PI uptake assay. WT etoposide vs. WT etoposide/Nec-1:p= 0.864, WT etoposide vs.MLKLKOetoposide:p= 0.1024, WT etoposide/Nec-1 vs.MLKLKOetoposide/Nec-1:p= 0.1791.MLKLKOetoposide vs.MLKLKOetoposide/Nec-1:p= 0.9628. Inb,c, andedata are shown as the mean ± SD (n= 3). Comparisons were performed using one-way ANOVA followed by the Tukey post-hoc test. **p< 0.01; NS: not significant. Source data are provided as a Source Data file. Fluorescence intensity (intensity × area) per cell was calculated using Image J software. In the integrin alpha5 trafficking assay, MEFs were treated with or without etoposide (10 µM), E64d (10 µg mL −1 ), and pepstatin (10 µg mL −1 ) for 12 h. Cells were then fixed for 12 h. Lysosomes were counterstained with an anti-Lamp1 antibody, and fluorescence intensity (intensity × area) per cell was calculated using Image J software. For FACS analysis, cells were transfected with VSVG–GFP, treated with or without etoposide (10 µM) in the presence of Q-VD-OPh (50 µM) at the permissive temperature (32 °C) for 60 min. Cells were then stained with an anti-VSVG antibody for 30 min at 4 °C without membrane permeabilization. After washing, the cells were stained with an Alexa fluor 633-conjugated secondary antibody for 30 min. After washing, cells were analyzed by flow cytometry. Data analysis was performed using BD FACSDiva and FlowJo software. Statistical analysis Results are expressed as the mean ± standard deviation (SD). Statistical analyses were performed using Excel and Prism 8 (GraphPad) software. Comparisons of two datasets were performed using unpaired two-tailed Student t -tests in Figs. 6 b, 8d , and Supplementary Fig. 22c . All other comparisons of multiple datasets were performed using one-way ANOVA followed by the Tukey post-hoc test. A p -value of <0.05 was considered to indicate a statistically significant difference between two groups. 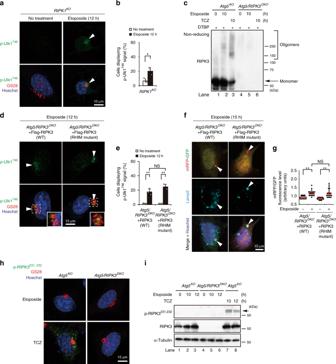Fig. 6: Different mechanisms of RIPK3 activation by etoposide and TCZ treatment. a,bRIPK1 is not involved in alternative autophagy.RIPK1KOcells were treated with or without etoposide (10 µM) for 12 h, and immunostained with anti-p-Ulk1746and anti-GS28 antibodies. Arrowheads indicate p-Ulk1746signals.bThe population of cells displaying p-Ulk1746signals was calculated (n≥ 100 cells).p= 0.025.cLack of RIPK3 oligomerization by etoposide treatment. The indicated MEFs were treated with or without etoposide or TCZ for 10 h. Cells were then incubated with 2 mM DTBP for 30 min. Nonreduced lysates were subjected to western blotting. Note the increase in oligomer bands and the decrease in the monomer band only by TCZ treatment.d–gNo requirement of the RHIM domain in etoposide-induced alternative autophagy. Similar experiments to Figs.1dand2bwere performed using Flag-RIPK3 (WT)-transfectedAtg5/RIPK3DKOMEFs and Flag-RIPK3 (RHIM mutant)-transfectedAtg5/RIPK3DKOMEFs. Representative images are shown ind. Magnified images are shown in the insets. Arrowheads indicate p-Ulk1746signals. Ine, the population of cells displaying p-Ulk1746signals was calculated (n≥ 100 cells).Atg5/RIPK3DKO+ RIPK3 (WT): no treatment vs. etoposide:p= 0.0004,Atg5/RIPK3DKO+ RIPK3 (WT) vs.Atg5/RIPK3DKO+ RIPK3 (RHIM mutant): etoposide:p= 0.0545. Representative images are shown inf. Arrowheads indicate mRFP–GFP red puncta. Ing, the extent of red puncta was indicated by the RFP/GFP ratio per cell (n= 20 cells). Red lines indicate the mean value.Atg5/RIPK3DKO+ RIPK3 (WT) vs.Atg5/RIPK3DKO+ RIPK3 (RHIM mutant) etoposide:p= 0.997.h,ip-RIPK3231,232is not induced in etoposide-induced alternative autophagy. The indicated MEFs were treated with etoposide (10 µM) or TCZ for 10 h. Inh, cells were immunostained with anti-p-RIPK3231,232and anti-GS28 antibodies. Ini, the expression of each protein was analyzed by western blotting. The p-RIPK3231,232signal (arrow) was observed in TCZ-treated MEFs, but not etoposide-treated MEFs. Inbande, data are shown as the mean ± SD (n= 3). Comparisons were performed using unpaired two-tailed Studentt-tests inbor using one-way ANOVA followed by the Tukey post-hoc testeandg. *p< 0.05; **p< 0.01; NS: not significant. Source data are provided as a Source Data file. Exact p values are described in figure legends, except that the values, using one-way ANOVA followed by the Tukey post-hoc test, are too large ( p > 0.9999) or small ( p < 0.0001) Statistics and reproducibility Repeated independent experiments per each panel with similar results are shown below. n = 1 (Figs. 1 a, 2a and Supplementary Figs. 1c, d , and 5). n = 2 (Figs. 1b, c , 3 a, b, 4 c, f, 5 d, 6 c, h, i, 7 a, e, 8a, c–f, h and 9c , Supplementary Figs. 1 a, b, 2a, 4b, 8a, 10a–d, 12a–d, 16b, 21a, 22a–c, 23c). 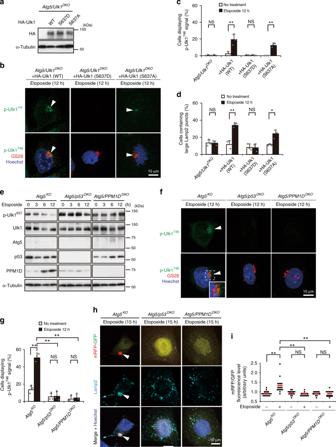Fig. 7: Requirement of p53/PPM1D-dependent dephosphorylation of Ulk1 at Ser637before the phosphorylation of Ulk1 at Ser746. aExpression of HA-Ulk1 mutants inAtg5/Ulk1DKOcells was confirmed by western blotting.b,cThe indicated MEFs were treated with or without etoposide (10 µM) for 12 h, and immunostained with anti-p-Ulk1746and anti-GS28 antibodies. Inb, representative images of p-Ulk1746and merged images are shown. Arrowheads indicate p-Ulk1746signals. Inc, the population of cells displaying p-Ulk1746signals was calculated (n≥ 100 cells).Atg5/Ulk1DKO+ HA-Ulk1 (S637A) no treatment vs. etoposide:p= 0.0012.dThe indicated MEFs were treated with or without etoposide (10 µM) for 12 h, and immunostained with anti-Lamp2 antibody. The population of cells containing large Lamp2 puncta was calculated (n≥ 100 cells). Representative images are shown in Supplementary Fig.17.Atg5/Ulk1DKO+ HA-Ulk1 (S637A) no treatment vs. etoposide:p= 0.0108.eEffects of p53 and PPM1D in the etoposide-induced modification of Ulk1. The indicated MEFs were treated with etoposide (10 µM) for the indicated times, and the expression of each protein was analyzed by western blotting.f,gRequirement of p53 and PPM1D for the etoposide-induced phosphorylation at Ulk1 Ser746. Similar experiments to Fig.1dwere performed. Inf, representative images of p-Ulk1746and merged images are shown. Arrowheads indicate p-Ulk1746signals. Ing, the population of cells displaying p-Ulk1746signals was calculated (n≥ 100 cells). p-Ulk1746signals were not observed inAtg5/p53DKOMEFs andAtg5/PPM1DDKOMEFs.Atg5/PPM1DDKO, no treatment vs. etoposide:p= 0.9933.h,iRequirement of p53 and PPM1D for etoposide-induced alternative autophagy. Similar experiments to Fig.2bwere performed using the indicated MEFs. Inh, representative images are shown. Arrowheads indicate mRFP–GFP red puncta. Ini, the extent of red puncta was indicated by the RFP/GFP ratio per cell (n= 20 cells). Red lines indicate the mean value.Atg5/p53DKO, no treatment vs. etoposide:p= 0.9201,Atg5/PPM1DDKO, no treatment vs. etoposide:p= 0.9987. Inc,d, andgdata are shown as the mean ± SD (n= 3). Comparisons were performed using one-way ANOVA followed by the Tukey post-hoc test. **p< 0.01; NS: not significant. Source data are provided as a Source Data file. n = 3 (Figs. 1 d–f, 2 b–g, 3 c–h, 4 a, b, d, e, g, h, 5 b, c, e, 6a–g , 7b–d , f–i, 8 b, 9 b, d, e, 10a, b and Supplementary Figs. 3a , b, 6 , 7a, b, 8b–f , 9a–c , 11a–d , 13a, b, 14a, b, 15a, b, 17a , 18a , b, 19a–d , 20a, b, 21b , 23a, b, d, e , 24a, b , 25a, b and 26a–d ). 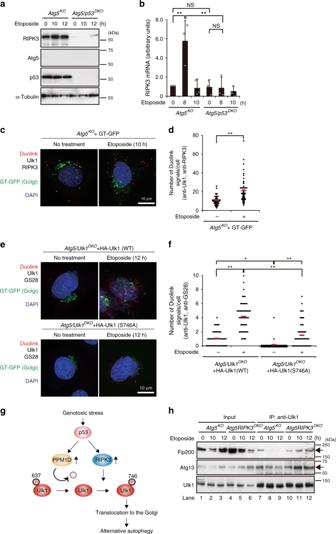Fig. 8: Mechanism of Ulk1746phosphorylation during etoposide treatment. a,bCrucial role of p53 in RIPK3 activation. The indicated MEFs were treated with etoposide (10 µM) for the indicated times. Ina, the expression of each protein was analyzed by western blotting. Inb, RIPK3 mRNA and 18S rRNA levels were analyzed using real-time PCR and their ratios were calculated. Values indicate the ratio to “Atg5KOtime 0”. Data are shown as the mean ± SD (n= 3).Atg5KO, no treatment vs. etoposide:p= 0.0029,Atg5KOvs.Atg5/p53DKOetoposide:p= 0.0023.c,dRIPK3–Ulk1 interaction occurs in the cytosol.Atg5KOMEFs were transfected with an expression vector for galactose transferase-fused GFP (GT-GFP); atrans-Golgi marker, and treated with or without etoposide (10 µM). The physical interaction between RIPK3 and Ulk1 was analyzed using Duolink reagents. All Duolink signals were localized in the cytosol. Ind, the number of Duolink signals were counted (n= 50 cells). Red bars indicate mean values.p= 7.4 × 10−7.e,fPhosphorylation-dependent translocation of Ulk1 to the Golgi.eThe indicated MEFs were transfected with GT-GFP and treated with or without etoposide (10 µM), and assayed with Duolink reagents using anti-Ulk1/anti-GS28 antibodies. Inf, the number of Duolink red signals were counted (n= 50 cells). Red bars indicate mean values.Atg5/Ulk1DKO+ HA-Ulk1 (WT) vs.Atg5/Ulk1DKO+ HA-Ulk1 (S746A), no treatment:p= 0.0137.gSchematic model of the RIPK3-dependent alternative autophagy. Genotoxic stress induces Ulk1 dephosphorylation at Ser637in a p53/PPM1D-dependent manner. The dephosphorylated Ulk1 is then phosphorylated at Ser746by RIPK3, and translocates to the Golgi, which results in alternative autophagy.hEffect of RIPK3 on the interaction of Ulk1 with Fip200 and Atg13. The indicated MEFs were treated with 10 µM of etoposide (10 µM). Cells were then lysed and immunoprecipitated with an anti-Ulk1 antibody. Immune complexes and total lysates (5.6% input) were analyzed by western blotting. Comparisons were performed using unpaired two-tailed Studentt-tests indor using one-way ANOVA followed by the Tukey post-hoc test inbandf. **p< 0.01; NS: not significant. Source data are provided as a Source Data file. 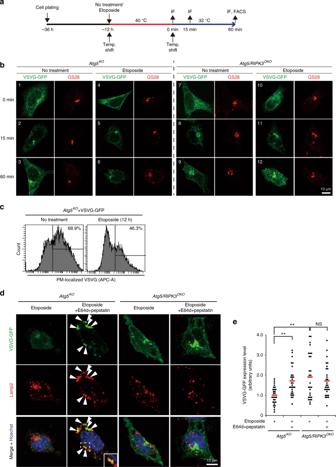Fig. 9: Effect of RIPK3 on the degradation of undelivered VSVG upon etoposide treatment. aSchematic diagram of the experiment. The VSVG–GFP was expressed inAtg5KOMEFs andAtg5/RIPK3DKOMEFs, and the cells were treated with or without etoposide (10 µM) at the restrictive temperature (40 °C) for 12 h. Cells were then shifted to the permissive temperature (32 °C), and fixed at the indicate times. Golgi was counterstained with an anti-GS28 antibody.bRepresentative images are shown. At 0, 15, and 60 min after the temperature shift, the location of VSVG–GFP and Golgi were analyzed.cReduction of PM-localized VSVG–GFP upon etoposide treatment. VSVG–GFP-expressingAtg5KOMEFs were or were not treated with etoposide, and at 60 min after the temperature shift, cells were stained with an anti-VSVG antibody for 30 min at 4 °C followed by the addition of an Alexa Fluor 633-conjugated secondary antibody for 30 min at 4 °C. After washing the cells, the amount of PM-localized VSVG–GFP was measured using flow cytometry.d,eVSVG–GFP-expressingAtg5KOMEFs andAtg5/RIPK3DKOMEFs were treated with etoposide (10 µM) in the presence of E64d/pepstatin. At 60 min after the temperature shift, cells were immunostained with an anti-Lamp2 antibody. Ind, representative images are shown. Arrowheads indicate autolysosomes containing VSVG–GFP. A magnified image of the areas within the dashed squares is shown in the insets. Ine, the amount of total VSVG–GFP (the level of fluorescence intensity in each cell) was measured using Image J (n= 30 cells in each experiment). Red bars indicate mean values.Atg5KOEtoposide vs. Etoposide with E64d/pepstatin:p= 0.0043,Atg5/RIPK3DKOEtoposide vs. Etoposide with E64d/pepstatin:p= 0.6495. Comparisons were performed using one-way ANOVA followed by the Tukey post-hoc test. **p< 0.01; NS: not significant. Source data are provided as a Source Data file. 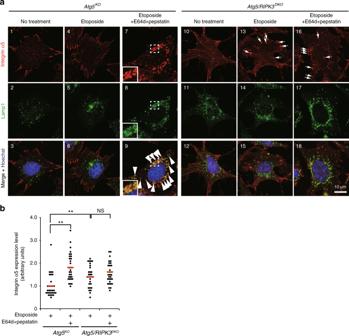Fig. 10: Requirement of RIPK3 for undelivered integrin α5 degradation upon etoposide treatment. TheAtg5KOMEFs andAtg5/RIPK3DKOMEFs were treated with or without etoposide (10 µM) in the presence of E64d/pepstatin for 12 h. Cells were immunostained with anti-Lamp1 and anti-integrin α5 antibodies. Ina, representative images are shown. Arrows and arrowheads indicate unusual cytoplasmic integrin alpha5 puncta and integrin α5 engulfed in autolysosomes, respectively. Magnified images of the areas within the dashed squares are shown in the insets. Note that etoposide generated unusual cytoplasmic integrin alpha5 puncta inAtg5/RIPK3DKOMEFs. Inb, the amount of total integrin α5 (the level of fluorescence intensity per cell) was measured (n= 30 cells in each experiment). Red bars indicate mean values.Atg5KOvs.Atg5/RIPK3DKOEtoposide:p= 0.0093,Atg5/RIPK3DKOEtoposide vs. Etoposide with E64d/pepstatin:p= 0.744. Comparisons were performed using one-way ANOVA followed by the Tukey post-hoc test. **p< 0.01; NS: not significant. Source data are provided as a Source Data file. Reporting summary Further information on research design is available in the Nature Research Reporting Summary linked to this article.